High photoresponsivity in an all-graphenep–nvertical junction photodetector Intensive studies have recently been performed on graphene-based photodetectors, but most of them are based on field effect transistor structures containing mechanically exfoliated graphene, not suitable for practical large-scale device applications. Here we report high-efficient photodetector behaviours of chemical vapor deposition grown all-graphene p – n vertical-type tunnelling diodes. The observed photodetector characteristics well follow what are expected from its band structure and the tunnelling of current through the interlayer between the metallic p - and n -graphene layers. High detectivity (~10 12 cm Hz 1/2 W −1 ) and responsivity (0.4~1.0 A W −1 ) are achieved in the broad spectral range from ultraviolet to near-infrared and the photoresponse is almost consistent under 6-month operations. The high photodetector performance of the graphene p – n vertical diodes can be understood by the high photocurrent gain and the carrier multiplication arising from impact ionization in graphene. Photodetectors (PDs) are nowadays recognized not only as a single-function device in detecting optical signals but also as a key component in the optoelectronic integration circuits that consist of light emitters, optical waveguides, PDs and electronic components on a single chip [1] , [2] . As major commercial products, GaN-, Si- and InGaAs-based PDs are available in the three important, UV, visible, and near-IR (NIR) subbands, respectively. Contrary to other two counterparts operated at room temperature (RT), InGaAs PDs should be cooled at 4.2 K for high detectivity. It would be advantageous to have a low-cost multicolour PD system showing high performance at RT over the broad spectral range from UV to NIR. Graphene has offered a broad spectral bandwidth potentially up to ~500 GHz and fast response time down to ~1.5 ps in PD applications [3] , [4] , [5] , [6] , [7] , [8] , [9] , but weak light absorption and low gain have limited key figures of merit such as quantum efficiency (QE), responsivity and noise equivalent power (NEP) of graphene PDs below 30%, 0.1 A W −1 and 200 n W Hz −1/2 , respectively [3] , [10] , [11] . Commercially available PDs show much better performances, but are not useful for transparent and flexible electronics and photonics. Thus, the demonstration of photodetection gain with graphene would be the basis for a variety of applications in flexible and transparent optoelectronics for biomedical imaging, remote sensing and optical communications. Previous studies of photocurrent (PC) in graphene have demonstrated photoresponse near metallic contacts [3] , [6] , [7] , [8] , at the interface between single-layer and bilayer regions [12] , at lateral-type p – n junctions [5] , [13] , [14] , or in the heterostructures with two-dimensional semiconductors [10] . The PC response was attributed to the presence of potential barriers at the metal contacts/the p – n junctions or across the heterostructures and could be modulated by sweeping gate voltages [3] , [4] , [6] , [10] , [13] . However, all these studies were based on field effect transistor structures containing mechanically exfoliated graphene, not suitable for practical large-scale device applications, and the magnitudes of PC were shown to be typically very weak compared with those in conventional semiconductor PDs owing to the low QE of graphene. Here we report a very practical chemical vapor deposition (CVD) graphene-based structure that works as a PD showing high performances in the UV–visible–NIR range. The PD structures permit a large PC flow by the tunnelling of charge carriers through the interlayer formed between the p - and n -graphene layers at higher n -doping concentrations [15] . Dark and photo I – V characteristics We prepared graphene p – n vertical tunnelling junctions for various doping concentrations of the n -type graphene layer by varying doping time ( t D ) in the benzyl viologen (BV) exposure while t D was fixed at 5 min in the AuCl 3 exposure. The devices were named as D1~D5 when t D in the BV exposure was 0.5, 1, 2, 3 and 4 min, respectively. The t D -dependent properties of the n - and p -graphene layers were analysed in detail [15] by using various structural, optical and electrical detection techniques [16] . 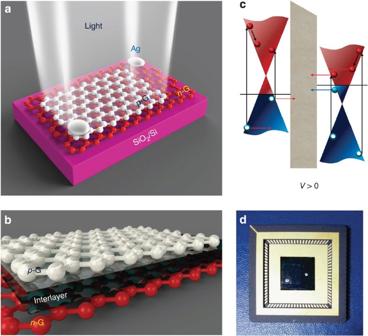Figure 1: Diagrams of schematics and band structure describing the PDs. Schematics of (a) a typical graphenep–ndiode for photodetection and (b) its magnified version showing an interlayer between metallicp- andn-graphene (p-G andn-G) layers. The diodes are illuminated with defocused light sources (xenon lamp or laser) with spot sizes that well match the device window of 5 × 5 mm2size. For the electrodes, Ag was used. (c) Band diagram of thep–nPD under forward (positive) bias. Red and white spots represent photoexcited electrons and holes, respectively, and lateral arrows indicate the transport directions of electrons and holes contributing to DCs and photocurrents. (d) A real image of a typical PD. Figure 1a shows a schematic of a typical graphene p – n vertical tunnelling junction for photodetection. Positive voltages were applied to the Ag electrode on p -graphene layer under forward bias. The dark current (DC)–voltage ( I – V ) curves are symmetric and linear in the forward/reverse directions with respect to zero voltage for D1–D3 devices, indicating no rectifying behaviours at the p – n junctions because of the negligible barrier at the boundary [15] . The I – V characteristics of these devices are almost not varied even under illumination at various photon wavelengths from 300 to 1,000 nm, as shown in Fig. 2a , resulting in no PC. Figure 1: Diagrams of schematics and band structure describing the PDs. Schematics of ( a ) a typical graphene p – n diode for photodetection and ( b ) its magnified version showing an interlayer between metallic p - and n -graphene ( p -G and n -G) layers. The diodes are illuminated with defocused light sources (xenon lamp or laser) with spot sizes that well match the device window of 5 × 5 mm 2 size. For the electrodes, Ag was used. ( c ) Band diagram of the p – n PD under forward (positive) bias. Red and white spots represent photoexcited electrons and holes, respectively, and lateral arrows indicate the transport directions of electrons and holes contributing to DCs and photocurrents. ( d ) A real image of a typical PD. 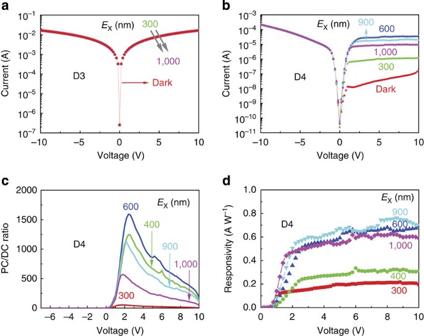Figure 2: Dark and photoI–Vcharacteristics and bias-dependent responsivity. I–Vcharacteristics of (a) D3 and (b) D4 devices under dark and illumination at various photon wavelengths from 300 to 1,000 nm. (c) On/off current ratios of D4 device as functions of bias voltage at various photon wavelengths from 300 to 1,000 nm. (d) Responsivities of D4 device as functions of forward bias at various photon wavelengths from 300 to 1,000 nm. Full size image Figure 2: Dark and photo I – V characteristics and bias-dependent responsivity. I – V characteristics of ( a ) D3 and ( b ) D4 devices under dark and illumination at various photon wavelengths from 300 to 1,000 nm. ( c ) On/off current ratios of D4 device as functions of bias voltage at various photon wavelengths from 300 to 1,000 nm. ( d ) Responsivities of D4 device as functions of forward bias at various photon wavelengths from 300 to 1,000 nm. Full size image For t D above 2 min (D4 and D5 devices), the DC is greatly reduced over the full range of bias voltage, with the current reduction being stronger under forward bias than under reverse bias, as shown in Fig. 2b (and Supplementary Fig. 1 ). The dark I – V curves show nonlinear properties with varying bias voltage, indicating rectifying behaviours. These anomalous I – V properties were attributed to actual formation of a structure like metal–insulator–metal/metal–semiconductor–metal diode due to strongly corrugated insulating or semiconducting interlayers formed between the metallic p - and n -graphene sheets at higher n -doping concentrations (see Fig. 1b ) and well explained based on the band structures of biased p – n junctions [15] ( Supplementary Fig. 2 ). The DC is of the order of 10 −8 A at a voltage of ~5 V for D4 device, indicating a very low leakage. Under illumination, large PC is obtained for forward bias, as shown in Fig. 2b , indicating a very high photosensitivity in this very simple structure. The photoresponse strongly depends on the photon wavelength. We find that the PC is of the order of μA for the bias voltages | V |>3 V, as shown in Fig. 2b , and observe a negligible change in the total current between before and after light illumination for negative bias. Since the total current is given by (DC+PC) and the contribution of PC to the total current is negligible, that is, DC>>PC for reverse bias, the total current is mainly determined by DC for negative bias, thereby making PC invisible for reverse bias. The D5 device shows lower photosensitivity owing to the higher DC ( Supplementary Fig. 1 ). The ratio of PC to DC or the on/off ratio of D4 device shows maximum intensities at bias voltages of around 2~3 V for various wavelengths ( λ ), as shown in Fig. 2c . The on/off ratio of D5 device shows similar bias voltage and λ dependences, but its magnitude is much smaller, regardless of bias voltage and λ ( Supplementary Fig. 1 ), resulting from larger DC. These I – V characteristics under dark as well as under illumination were almost not varied by using Au as an electrode ( Supplementary Fig. 3 ). The rectifying behaviour of the DC can be understood from the available density of states for tunnelling between p - and n -type graphene [15] ( Supplementary Fig. 2 ). For positive bias the current is severely suppressed due to minimizing of joint density of states for tunnelling. When the graphene p – n junction is illuminated by laser light, electrons in valence band are excited to conduction band, producing electron–hole pairs. In the presence of photoexcitation both electrons and holes contribute to the PC. Especially, in our graphene p – n junction the tunnelling current by holes is more significant than the current by electrons for a positive bias because the tunnelling of electrons is restricted by the joint density of states, but there is no restriction for hole tunnelling, as shown in Fig. 1c . In graphene, since the relaxation due to the carrier–phonon scattering is much slower than that due to the carrier–carrier scattering [17] , [18] , a single photon produces multiple electron–hole excitations by impact ionization induced by a hot electron [19] , [20] . Thus, the carrier multiplication enhances the PC. The PC dominates over the DC when the DC is small for positive bias while the PC is not visible when the DC is very large for reverse bias, as shown in Fig. 2b and Supplementary Fig. 1 . Photosensitivity and detectivity We also prepared graphene p – n vertical tunnelling junctions for various doping concentrations of the p -type graphene layer by varying t D in the AuCl 3 exposure while t D was fixed at 3 min in the BV exposure, and found that the device characteristics were optimized at t D =5 and 3 min for AuCl 3 and BV exposures (D4 device), respectively ( Supplementary Fig. 3 ). We characterized D4 and D5 devices in detail by measuring several figures of merit essential for the evaluation of a PD. Figure 2d shows responsivity (the electrical current response to the incident optical power, R i ) of D4 device, measured as a function of bias voltage for various λ . There are no big variations in R i above around 2~3 V irrespective of λ . R i at λ ~900 nm reaches ~0.7 A W −1 at 6 V. At λ ~400 nm, R i is reduced to ~0.3 A W −1 because less light was absorbed by the device. 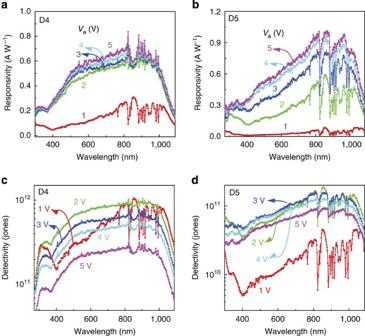Figure 3: Spectral responsivity and detectivity. Spectral responsivities of (a) D4 and (b) D5 devices at different forward-bias voltages from 1 to 5 V. Spectral detectivities of (c) D4 and (d) D5 devices at different forward-bias voltages from 1 to 5 V. Figure 3a,b compares the spectral R i of D4 and D5 devices for bias voltages from 1 to 5 V. There are small variations in the spectral R i of D4 device for bias voltages ≥2 V. In contrast, the D5 shows a gradual increase in the spectral R i with increasing the bias voltage up 5 V; in other words, the R i is more sensitive to the variation of the bias voltage in D5 device ( Supplementary Fig. 1 ). The R i of D5 device in the UV range (300–400 nm) reaches ~0.4 A W −1 at 6 V, ( Supplementary Fig. 1 ) while that in the NIR range (700–950 nm) is as high as ~1.0 A W −1 , as shown in Fig. 3b . These R i values are higher than (or comparable to) those reported for commercially available Si and InGaAs PDs (~0.5 and ~0.9 A W −1 , respectively) [21] , [22] . The DC decreases with decreasing temperature ( T ), resulting in higher on/off ratio and R i under forward bias at lower T ( Supplementary Fig. 4 ). Figure 3: Spectral responsivity and detectivity. Spectral responsivities of ( a ) D4 and ( b ) D5 devices at different forward-bias voltages from 1 to 5 V. Spectral detectivities of ( c ) D4 and ( d ) D5 devices at different forward-bias voltages from 1 to 5 V. Full size image The QE can be calculated by normalizing the number of photogenerated carriers by the number of absorbed photons for any given λ . In both D4 and D5 devices, the magnitude of the QE increases with increasing V ; however, this increase is not linear ( Supplementary Fig. 5 ). Furthermore, the QE is not spectrally uniform and shows a relatively clear peak around ~500 nm in D4 device, but the QE peak is not pronounced in D5 device. By considering the spectral R i in Fig. 3a,b , it is noted that a strong enhancement is especially reflected in high-energy side of QE, consistent with the fact that the absorption spectra of doped graphene sheets are peaked at high energies ( Supplementary Fig. 6 ). The QEs of D4 and D5 devices are over 100% at bias voltages of 4 and 5 V, which will be explained later in detail based on the transient PC data. A key figure of merit for a PD is the NEP. This parameter is defined as the amount of incident light power that generates a PC equal to the noise current. The NEP can be expressed as [23] : NEP=( I n 2 ) 1/2 / R i where I n 2 is the time-averaged square of the total noise current and can be estimated by integrating spectral density of noise power ( Supplementary Fig. 7 ). Then, the NEP can be calculated by using the spectral R i data in Fig. 3a,b ; ( Supplementary Fig. 7 ). Another parameter used to characterize the performance of PDs is the detectivity ( D* ), which is related to NEP by the expression: D* =( A Δ f ) 1/2 /NEP. Here A is the effective area (~0.5 × 0.5) of the detector in cm 2 and Δ f is the electrical bandwidth in Hz. The D* of both devices increases with increasing the bias up to ~2 V, but above ~2 V it decreases over almost full range of λ , as shown in Fig. 3c,d . The maximum D* at ~2 V is closely related to the largest on/off ratio at 2~3 V, as shown in Fig. 2c . Relatively poor D* for D5 device may be due to high DC ( Supplementary Fig. 1 ). Owing to its fairly ‘flat’ spectrum, the D* of D4 device remains high on both the blue (4.0 × 10 11 cm Hz 1/2 W −1 or Jones at 400 nm) and the NIR (1.0 × 10 12 Jones at 900 nm) ends of the spectrum at 2 V. The D* value of D5 device (for example, 4.8 × 10 10 and 1.2 × 10 11 Jones at 400 and 900 nm, respectively, for a bias voltage=3 V) is smaller than that of device D4, but the response of D5 device is more spectrally uniform for bias voltages ≥2 V. These values are comparable to those of Si and InGaAs PDs (~4 × 10 12 and >10 12 Jones (4.2 K), respectively) [24] . 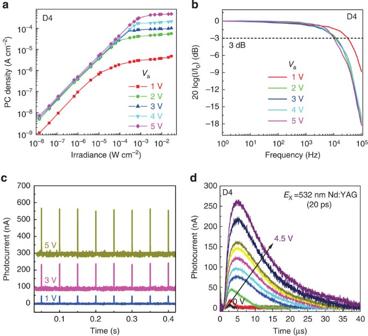Figure 4: Linearity and time response. (a) Irradiance-dependent PC densities of D4 device at different forward-bias voltages from 1 to 5 V. (b) Frequency-dependent PC response of D4 device at different forward-bias voltages from 1 to 5 V. (c) Repeated PC response switching of D4 device at different forward-bias voltages from 1 to 5 V. (d) Transient PCs of D4 device at different forward-bias voltages from 0 to 4.5 V in 0.5 V step. The PC switching and transient behaviours were measured by using 20 ps, 20 Hz Nd:YAG laser pulses at 532 nm. Linearity and time response Figure 4a shows PC density ( J PC ) of D4 device versus incident light power of a 532-nm laser line at various bias voltages, which was obtained at a modulation frequency of 30 Hz. The J PC strongly depends on the illumination power. Neutral density filters were used to change the incident light power ( P ). For lower light powers spanning three orders of magnitude, the J PC increases linearly with P , and after a threshold power it deflects from the linear relationship. The threshold power increases with increasing the bias voltage, as shown in Fig. 4a . The J PC in the linear region can be expressed by a simple power law: J PC P α , where 0.95< α <1.08 in this work. The linear increase of the PC density is attributed to the linear photogeneration of electron–hole pairs. However, at high powers the photogenerated electron–hole pairs can recombine before reaching electrodes possibly because of their trapping at the surface/interface states [25] , resulting in the saturation of the PC density at high powers. Figure 4: Linearity and time response. ( a ) Irradiance-dependent PC densities of D4 device at different forward-bias voltages from 1 to 5 V. ( b ) Frequency-dependent PC response of D4 device at different forward-bias voltages from 1 to 5 V. ( c ) Repeated PC response switching of D4 device at different forward-bias voltages from 1 to 5 V. ( d ) Transient PCs of D4 device at different forward-bias voltages from 0 to 4.5 V in 0.5 V step. The PC switching and transient behaviours were measured by using 20 ps, 20 Hz Nd:YAG laser pulses at 532 nm. Full size image Another figure of merit for PDs is the linear dynamic range (LDR) or photosensitivity linearity (typically quoted in dB). LDR is given by LDR=20 log ( J* PC / J d ), where J* PC is the PC density measured at a light intensity of 1 mW cm −2 and J d is the DC density. The ratio of full-well capacity of today’s complementary metal-oxide-semiconductor image sensors to the number of dark electrons limits dynamic range to about three orders of magnitude in intensity (conventionally expressed as 60 dB in imaging); in other words, more than 60 dB is required for the imaging application of PDs. As calculated from the J PC versus irradiance curve, as shown in Fig. 4a , the LDR of D4 device is ~93 dB (~85 dB for D5 device; Supplementary Fig. 8 ), which is comparable to that of Si PDs (~120 dB) and significantly higher than that of InGaAs PDs (~66 dB) [24] , [26] . The LDR increases with increasing the bias voltage ( Supplementary Fig. 8 ). Figure 4b shows the frequency ( f )-PC response of D4 device. The PC response is independent of f at f <~3 × 10 4 Hz at 1 V, but begins to decrease at f ≥~3 × 10 4 Hz. This transition corresponds to the minimum carrier lifetime required for photocarriers generated in the n (or p ) region to tunnel into the p (or n ) region. The 3-dB frequency decreases with increasing the forward bias, as shown in Fig. 4b ( Supplementary Fig. 8 for D5 device), because of an increase in tunnelling time with increasing electric field in the interlayer region between the p- and n -graphene sheets. The linearity of R i with the light power is also enhanced at higher bias voltages ( Supplementary Fig. 8 ). Figure 4c shows PC response switching at various bias voltages by using 20 Hz, 532 nm laser pulse. The laser was focused onto the PD devices with a spot size of ~5 × 5 mm 2 . Within 40 μs after the light is turned off, the current reaches the initial DC value. The PC switching behaviours are very regular for each pulse, almost irrespective of the bias voltage. The D5 device shows similar switching behaviours ( Supplementary Fig. 9 ). To probe the charge-transfer dynamics, transient PCs were recorded at much smaller timescale for various bias voltages, as shown in Fig. 4d ; ( Supplementary Fig. 9 for D5 device). The turn-on transient response is characterized by a relatively fast increase in the PC during several tens of ns, followed by a relatively slow decay to a steady-state value during several μs, which is attributed to electron–hole recombination. The rise time is the time required for generation of carriers in the n or p region and tunnelling in the p – n junction, and is dependent on the width of the interlayer. As reported before [27] , the charge state of the BV molecules in the interlayer can be changed by UV illumination, thereby changing the film transmittance, but the response time is approximately several tens of seconds, much longer than the decay time in our work. Instead, considerable amount of trap states can be formed at the interlayer/ p- and n -graphene sheets, thereby inducing multiple trappings of carriers, resulting in slower decay of photoexcited carriers in the graphene p – n device, compared with the field effect transistor structures containing pristine graphene [3] , [9] . The decay time as well as the rise time increases with increasing the bias voltage for the D4 and D5 devices ( Supplementary Fig. 9 ) but these behaviours do not seem to be relevant to the RC time constant of the p – n structures, showing a decrease with the increase of the bias voltage ( Supplementary Fig. 9 ). The switching time is estimated to be tens of μs depending on the bias voltage. The PDs should be reliable under long-term operations. Therefore, we studied long-term stabilities of the PD performance by measuring R i at various voltages for 6 months in air, and found the R i was consistent under 6-month operations regardless of bias voltage ( Supplementary Fig. 10 ). It should be noted that the measured QEs are the effective ones, that is, η eff = ηG , where η and G are the QE and the internal gain of the device, respectively [28] . We expect the D4 and D5 devices can show remarkably high η values owing to a carrier multiplication of ~2.5 in graphene [19] , the doping-enhanced absorption reaching up to ~10% in each n - or p -graphene layer [15] and the p – n graphene double-layer structure. In addition, extremely high gain is expected in D4 and D5 devices because the gain is given by the ratio of the carrier lifetime ( τ ) to the transit time ( t ) across the electrodes, G~ τ /t , and from the transient PC the lifetime of electron–hole pair is estimated to be an order of μs ( Supplementary Fig. 9 ). The electron–hole pairs are produced within several tens of ns ( Supplementary Fig. 9 ) on a light pulse and in the vertical junction they transit to the opposite electrode immediately from the place where they are generated. Thus, the current gain in the vertical junction can exceed an order of 10 2 . Combining these two effects, it is possible to obtain effective QEs almost over 100% in D4 and D5 devices. However, in the lateral graphene p – n [5] , [13] , [14] or the graphene–metal [3] , [4] junctions the gain is expected to be very low because the spacing between the electrodes is typically an order of μm. Thus, it may be possible to get the high effective QE only in vertical p – n junctions. These results demonstrate that the performance parameters of all-graphene PDs based on their p – n vertical junctions are comparable to or even better than commercially available PDs made of Si or compound semiconductor materials. The achievement of high-performance all-graphene PDs implies that graphene can be used in a variety of possible transparent and flexible optoelectronics applications and will open exciting opportunities not only for the creation of single-function PDs with wide spectral range but also for the fabrication of high-resolution PD arrays for imaging, sensing and optical communications. Doping of graphene The graphene films were prepared by CVD and subsequently transferred to the 300-nm SiO 2 / p -type Si wafers. Gold chloride (AuCl 3 ) powder and 1,1′-dibenzyl-4,4′-bipyridinium dichloride (BV 2+ ) (Sigma-Aldrich) were used for p - and n -type dopants, respectively. AuCl 3 powder was dissolved in nitromethane to yield 10 mM solution and BV 2+ was reduced in a biphasic solution of water/toluene to prepare 10 mM BV 0 solution [15] . For the doping of graphene, the dopant solution was dropped on the whole surface of graphene sheet and after some time (this time was defined as doping time, t D ) elapsed, it was spin coated at 2,000 r.p.m. for 1 min. The t D was varied to change doping concentration. Fabrication of p – n devices For the formation of graphene p – n PD, a solution of BV was first dropped and spin coated on the 10 × 10-mm 2 graphene/SiO 2 / p -type Si wafer, and then annealed at 100 °C for 10 min to make graphene uniformly n -type. The annealing temperature was optimized through repeated experiments for the good quality-doped graphene. Subsequently, a 5 × 5-mm 2 bare graphene was transferred on ~1/4 area of the n -graphene/SiO 2 / p -type Si wafer, a solution of AuCl 3 was dropped and spin coated on the surface of graphene, and similarly annealed. As a result, the graphene p – n vertical junction was formed on the ~1/4 area of the SiO 2 / p -type Si wafer. One millimetre diameter Ag or Au electrodes were deposited on the top of both n - and p -graphene layers to complete the graphene p – n PD. Measurements I – V measurements to characterize the electrical behaviours of graphene p – n PDs were carried out using a Keithley 2,400 source meter controlled by a LabView program. The DC noise under forward bias was measured with a dynamic signal analyser (Agilent 35670A) coupled to a low-noise current preamplifier (Stanford Research SR570) in the frequency range of 1 Hz~5 kHz. During the measurements, the PDs were mounted in a dark, electrically shielded and optically sealed chamber on the optical table to reduce vibrational noise. The spectral photoresponse was detected in the 300–1,100 nm wavelength range. For this purpose, we used a 450-W xenon light source and a 0.25-m grating monochromator (Newport Cornerstone 260 1/4 m monochromator). The incident light intensity was monitored by a motorized variable wheel attenuator and a Newport calibrated UV-enhanced silicon photodiode. The power density of the incident light on the sample surface was about 1~320 μW cm −2 depending on the wavelength in the range of 300~1,100 nm. A 532-nm monochromatic light from a diode laser was used for studying the photosensitivity linearity with light power. The light was modulated with a mechanical chopper (Stanford Research Systems) at 30 Hz, and the PC response at various bias voltages was recorded with a Signal Recovery 7,265 DSP lock-in amplifier. Optical neutral density filters were used to vary the light intensity from nW up to 7.2 mW. (maximum power: 90 mW). For frequency dependence of the PC, the graphene p – n PD was illuminated by a Thorlabs 50 μW, 530 nm light-emitting diode array with an Instek SFG-830 30 MHz function generator used to supply a constant or modulated bias to the light-emitting diodes. The PC response was measured with an SR530 lock-in amplifier coupled to a current preamplifier (Stanford Research SR570) in the frequency range of 1–100 kHz. Transient PC studies were conducted using laser pulses from the Nd:YAG laser (532 nm wavelength, 20 ps duration and 20 Hz repetition rate, generated by a Continuum Leopard-D20 Nd:YAG laser), which were focused onto the PD devices with a spot size of ~5 × 5 mm 2 . A laser power meter (Laser probe, Rj-760) was used to measure the average power of the laser pulses. The laser pulse temporal profiles and transient PC were monitored with the 50 ohm terminated, 500 MHz bandwidth digital oscilloscope (Tektronix DPO 4054). All measurements were performed in a dark, shielded enclosure under vacuum at RT. How to cite this article: Kim, C. O. et al. High photoresponsivity in an all-graphene p – n vertical junction photodetector. Nat. Commun. 5:3249 doi: 10.1038/ncomms4249 (2014).